Improving battery safety by early detection of internal shorting with a bifunctional separator Lithium-based rechargeable batteries have been widely used in portable electronics and show great promise for emerging applications in transportation and wind–solar-grid energy storage, although their safety remains a practical concern. Failures in the form of fire and explosion can be initiated by internal short circuits associated with lithium dendrite formation during cycling. Here we report a new strategy for improving safety by designing a smart battery that allows internal battery health to be monitored in situ . Specifically, we achieve early detection of lithium dendrites inside batteries through a bifunctional separator, which offers a third sensing terminal in addition to the cathode and anode. The sensing terminal provides unique signals in the form of a pronounced voltage change, indicating imminent penetration of dendrites through the separator. This detection mechanism is highly sensitive, accurate and activated well in advance of shorting and can be applied to many types of batteries for improved safety. The energy and power density of electrochemical rechargeable batteries has increased significantly in recent years [1] , [2] , [3] , [4] . Meanwhile, safe operation of these high-energy devices has become a stringent requirement, especially for applications in large-scale renewable energy storage and electric grid, electric drive vehicles, airplanes and next-generation portable electronics [1] , [2] , [4] , [5] , [6] , [7] . For both lithium-ion and lithium metal rechargeable batteries, safety issues are often associated with the formation of dendritic lithium on the negative electrode [8] . In the lithium metal rechargeable battery, lithium dendrites gradually grow on the surface of the lithium metal electrode during each discharge–recharge cycle [7] . These dendrites can penetrate through the polymer separator to form a short circuit between the positive and negative electrodes [9] , which can initiate exothermic reactions between the electrodes and the flammable organic electrolyte [10] , [11] . The excess of heat released in these reactions often induces fire and even explosions. Owing to the inherent instability of lithium metal deposition, research shifted to lithium-ion-based batteries during the 1980s (refs 1 , 2 , 4 ). Current commercial lithium-ion batteries using graphite as a negative electrode exhibit an approximately tenfold lower specific charge capacity but safer operation compared with lithium metal electrodes; however, despite this development, lithium dendrite formation has not been entirely inhibited in graphite anodes either, especially when cycled at high current densities, in overcharge conditions, or at low temperatures [8] , [12] , [13] , [14] , [15] . In the last few decades, considerable efforts have been devoted to suppressing dendrite growth by improving electrode materials [16] , [17] , electrolyte additives [18] , [19] , separators [9] , [20] , [21] , [22] , [23] and battery management systems [8] with some success, although they still do not solve the problem. Typical examples are the re-engineering of the surface morphologies and coating processes of the electrodes [16] , [17] , [24] , modification of the electrolyte solvent and solute [18] , [19] , [25] , [26] , [27] , [28] , incorporation of hard ceramic coatings onto the porous polymer separator [5] , [20] , [21] , [23] and theoretical modelling [29] , [30] of the mechanisms leading to dendrite formation. Unfortunately, despite intense study for several decades, it seems nearly impossible to completely eliminate dendrite formation with current technologies, as the lithium re-deposition process is inherently non-uniform and predisposed to formation of dangerous lithium dendrites. Herein, instead of suppressing dendrite formation, we report a smart battery that employs an alternative strategy of detecting dendrite growth before it forms a complete internal short circuit. The battery can then be taken offline before any accidents occur. The early detection of dendrite growth inside lithium batteries is achieved through a bifunctional separator design employing a third sensing terminal to monitor internal battery conditions. Material design A schematic representation of our proposed smart battery concept is shown in Fig. 1 . Traditional battery cells always consist of a positive and a negative electrode (both sources of chemical reactions) separated by an electrolyte solution containing dissociated salts to enable ion transfer between the two electrodes. During repeated charging of lithium-based batteries, lithium is unevenly electroplated onto the lithium anode surface forming dendrites, which eventually penetrate the separator and make electrical contact with the cathode, leading to internal short circuits ( Fig. 1a ). The traditional battery separator is an electronic insulating layer with a porous structure made of inert polymers; they are not effective in blocking the overgrowth of dendrites. In our design, we change the separator to a polymer–metal–polymer triple layer configuration ( Fig. 1b ). It is noteworthy that although a thin and porous conducting metal has been introduced as an intermediary layer, the sandwiched membrane maintains electronic insulation between the two electrodes and still functions effectively as a separator. We call it ‘bifunctional separator’, as it provides both the traditional separator function and a new voltage-sensing function. Owing to the electrochemical potential difference, the voltage between the intermediary metal and the anode can be monitored. During battery cycling, dendrites will form on the anode and grow until they inevitably reach the intermediate metal layer before puncturing through the whole separator. When a dendrite connects the metal layer with the anode, a voltage drop between them can be detected immediately. At this stage, the dendrite has not caused internal shorting between anode and cathode. On detection of this distinctive signal of abnormal function, the battery can be safely removed from service, effectively preventing fire and explosion, which can be the result if the short circuit reaction is allowed to proceed uncontrolled. 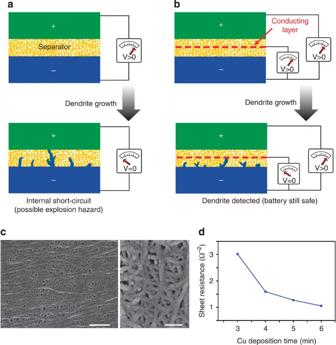Figure 1: Schematic of the smart battery design and fabrication. (a) Dendrite formation in a traditional lithium battery where complete penetration of the separator by a lithium dendrite is only detected when the battery fails due to an internal short circuit andVLi-Lidrops to zero. (b) In comparison, a lithium battery with a bifunctional separator (consisting of a conducting layer sandwiched between two conventional separators) where the overgrown lithium dendrite penetrates into the separator and makes contact with the conducting copper layer, giving rise to a drop inVCu-Lias warning of impending failure due to an internal short circuit. However, the full battery remains safely operational with non-zero potential. (c) Scanning electron microscopy images of commercial polymer separator coated with a 50-nm copper layer, which preserves the separator’s porous surface morphology. Scale bars 1 μm (left of panel) and 200 nm (right of panel). (d) The sheet resistance of separator after copper deposition for varying times. Figure 1: Schematic of the smart battery design and fabrication. ( a ) Dendrite formation in a traditional lithium battery where complete penetration of the separator by a lithium dendrite is only detected when the battery fails due to an internal short circuit and V Li-Li drops to zero. ( b ) In comparison, a lithium battery with a bifunctional separator (consisting of a conducting layer sandwiched between two conventional separators) where the overgrown lithium dendrite penetrates into the separator and makes contact with the conducting copper layer, giving rise to a drop in V Cu-Li as warning of impending failure due to an internal short circuit. However, the full battery remains safely operational with non-zero potential. ( c ) Scanning electron microscopy images of commercial polymer separator coated with a 50-nm copper layer, which preserves the separator’s porous surface morphology. Scale bars 1 μm (left of panel) and 200 nm (right of panel). ( d ) The sheet resistance of separator after copper deposition for varying times. Full size image Material synthesis and electrode fabrication To demonstrate the proposed battery protection mechanism experimentally, we fabricated the bifunctional separator by simply stacking two conventional porous polymer separators with 12 μm thickness, one of which was pre-deposited with a 50-nm-thick copper layer by magneto sputtering without additional heating, as the separator is sensitive to heat (see Supplementary Fig. 1 and fabrication process in Methods). We chose copper to serve as the metal in the triple layer configuration, as it is stable in the electrolyte and has a sufficiently large difference in electrochemical potential with Li, although other metals are also viable. When compared with traditional separators, the bifunctional separators have five key properties, which are important for smart batteries: (1) thin metal deposition by magneto sputtering does not alter the macroscopic morphology of the separator as shown in the scanning electron microscopy image in Fig. 1c . The thickness of the metal layer is <1% of the total thickness of the separator, which does not affect the mechanical strength of the separator, a practical consideration for construction of the battery cell. (2) The metal coating side of the separator becomes highly conducting in plane for voltage sensing. As shown in Fig. 1d , the sheet resistance is very low <3 Ω −2 . (3) Across the separator, the electrical resistance remains very high. The directionality of the sputtering process and the three-dimensional porous structure of the polymer separator allows metal to be deposited only on the outer surface without permeating the interior of the membrane as shown in the cross-sectional view of the separator ( Supplementary Fig. 2 ), thus ensuring electrical insulation of the stacked trilayer separator. As shown in Supplementary Fig. 3 , the electrical resistance of the separator before and after metal coating remains the same in the very high range of ~10 12 Ω. (4) The sputtering process does not affect the ionic conductivity of the separator. Figure 1c presents the surface morphology of the metal-coated separator. Clearly, the highly porous structure of the separator is preserved after metal deposition of such a thin layer without hindering lithium ion transfer across the separator. According to electrochemical impedance spectroscopy measurements, the separator exhibits excellent ionic conductivity of ~0.3 mS cm −1 before and after different thicknesses of metal coating ( Supplementary Figs 4 and 5 ). The metal coating is mechanically flexible. In cell manufacturing, the separator undergoes various forces and deformations due to the rolling and folding processes before it is packed inside the battery pouch or casing. Therefore, the mechanical flexibility and stability of the thin metal interlayer inside the bifunctional separator is important for practical battery assembly. Our experimental results ( Supplementary Figs 5–8 ) show that the thin metal coating is strongly adhered to the polymer separator and, furthermore, it exhibits superior mechanical flexibility, indicating that its integrity can be maintained through the production cycle. Dendrite detection The trilayer separator is assembled into lithium batteries with a third terminal connected to the copper layer. During standard operation of a lithium metal battery, dendrite growth is very slow and usually requires long time scales to completely penetrate the separator. To examine the formation of lithium dendrites within reasonable time frames, we used two lithium metal electrodes with high galvanostatic current densities to accelerate the growth of dendrites. As shown in Fig. 2a , for a battery with a traditional separator, the voltage between the two electrodes ( V Li-Li ) was initially 400 mV due to overpotential before sharply dropping to 200 mV when charged at a current density of 4.0 mA cm −2 . V Li-Li then gradually increased to 500 mV due to impedance increase during the formation of an insulating solid electrolyte interphase (SEI) layer. Further charging initiated a sudden drop of V Li-Li to nearly zero, which correlates to the appearance of a short circuit caused by penetration of the separator as has been previously reported [31] . The small non-zero voltage results from the electrical resistance of the lithium dendrite bridge between the two electrodes. 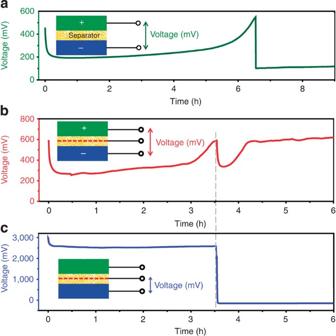Figure 2: Experimental demonstration of dendrite detection. (a) Voltage profile of a Li/Li battery with a conventional separator under accelerated charging at a current density of 4 mA cm−2. Just after initiation of charging, the voltage drops sharply due to over potential until it reaches its optimal value. The voltage then gradually increases over the following several hours due to SEI formation. After ~6.5 h, the battery is shorted as a result of dendrite growth withVLi-Lidropping to almost zero. (b) Voltage profile of a Li/Li battery with a bifunctional separator under accelerated charging at a current density of 4 mA cm−2, whereVLi-Li(red) is monitored. For a Li/Li battery with conventional separator, the voltage shows an initial sharp drop due to overpotential. The potential then gradually increases to 500 mV as a result of SEI formation. After ~3.5 h, the lithium dendrite reaches the copper coating on the separator causing the full cell potential to abruptly drop to 250 mV due to a decrease in impedance. However, the full cell remains safely operational with non-zero voltage after the dendrite is detected. (c) Voltage profile of the same Li/Li battery with a bifunctional separator under accelerated charging as inb, whereVCu-Li(blue) is monitored. Corresponding to the dip inVLi-Liwhen the lithium dendrite makes contact with the copper interlayer,VCu-Lidrops to ~0 V as the potential difference of 3,000 mV between the two metals is dissipated on contact. Figure 2: Experimental demonstration of dendrite detection. ( a ) Voltage profile of a Li/Li battery with a conventional separator under accelerated charging at a current density of 4 mA cm −2 . Just after initiation of charging, the voltage drops sharply due to over potential until it reaches its optimal value. The voltage then gradually increases over the following several hours due to SEI formation. After ~6.5 h, the battery is shorted as a result of dendrite growth with V Li-Li dropping to almost zero. ( b ) Voltage profile of a Li/Li battery with a bifunctional separator under accelerated charging at a current density of 4 mA cm −2 , where V Li-Li (red) is monitored. For a Li/Li battery with conventional separator, the voltage shows an initial sharp drop due to overpotential. The potential then gradually increases to 500 mV as a result of SEI formation. After ~3.5 h, the lithium dendrite reaches the copper coating on the separator causing the full cell potential to abruptly drop to 250 mV due to a decrease in impedance. However, the full cell remains safely operational with non-zero voltage after the dendrite is detected. ( c ) Voltage profile of the same Li/Li battery with a bifunctional separator under accelerated charging as in b , where V Cu-Li (blue) is monitored. Corresponding to the dip in V Li-Li when the lithium dendrite makes contact with the copper interlayer, V Cu-Li drops to ~0 V as the potential difference of 3,000 mV between the two metals is dissipated on contact. Full size image In a battery with this trilayer separator design, the voltage between the intermediate copper layer and lithium electrode ( V Cu-Li ) is also monitored while charging the battery at the same current density (4.0 mA cm −2 ). As illustrated in Fig. 2c , initially V Cu-Li is ~3,000 mV, mainly due to the electrochemical potential difference between lithium and copper. After 3.5 h of charging, a sharp drop in V Cu-Li appears to indicate that the lithium dendrite has made contact with the copper layer. The physical contact dissipates the 3,000 mV potential difference as the lithium electrode is now electrically connected with the copper interlayer; simultaneously, a change in V Li-Li (as illustrated in Fig. 2b ) from 500 mV to around 250 mV was detected. The temporary decrease of the potential is mainly due to the reduction of cell impedance on electrical connection of the copper layer with the lithium electrode by the lithium dendrite. This contact opens up the copper surface for lithium deposition, resulting in decreased distance between the two lithium electrodes. A gradual rise in potential occurs a second time due to renewed SEI formation on the newly deposited lithium metal at the copper surface. The two lithium electrodes, however, remain electrically isolated from one another, indicating that the battery is still safely operational at this stage. The sudden drop in V Cu-Li at 3.5 h can be recognized as a safety alarm, indicating lithium dendrite penetration through half of the separator. It is worth mentioning that by simply varying the thickness ratio between the two separator layers, the critical point at which an alarm is generated can be tuned to indicate 25%, 50%, 75%, or any degree of separator penetration by a lithium dendrite. The dendrite alarm mechanism is further confirmed by in situ observation of dendrite growth inside a battery. To examine the battery operation in an optical microscope, we fabricated a battery device sealed in a transparent pouch cell with electrolyte, which was constructed by placing two thin lithium metal tips beside a polymer separator with copper deposited on one side ( Supplementary Fig. 9 ). 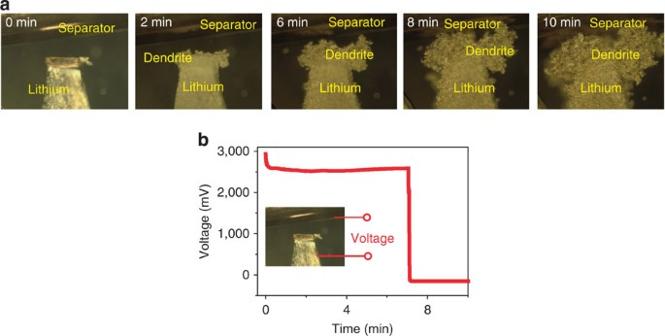Figure 3:In-situobservation of dendrite growth on lithium electrode. (a) A lithium anode and separator-wrapped lithium counter electrode with copper conductive layer facing the lithium anode housed in a glass cell forin-situoptical microscopy observation. During charging of the cell, non-uniform deposition of lithium onto the lithium electrode leads to mossy dendrite formation and growth on the surface. (b) Voltage profile of the device. The lithium dendrites make contact with the conductive copper layer on the separator at about 6–8 min, giving rise to a 3 V drop inVCu-Li, as the potential difference between copper and lithium is dissipated on contact. Figure 3 shows lithium being continuously electroplated onto the lithium electrode surface during accelerated electrochemical charging, consequently inducing dendrite formation and growth. The voltage between the copper layer and the lithium tip on the separator, V Cu-Li , is monitored during this process. The value is initially measured to be around 3,000 mV, representing the potential difference between lithium and copper. As lithium is continuously electrodeposited, the dendrite grows across the electrode gap until it makes contact with the copper layer on the separator ( Supplementary Fig. 10 ), and the potential between lithium and copper suddenly drops to ~0 V between 6 and 8 min of charging. The dendrite detection mechanism has also been demonstrated in a LiCoO 2 /Li battery system ( Supplementary Fig. 11 and Supplementary Note 1 ). Figure 3: In-situ observation of dendrite growth on lithium electrode. ( a ) A lithium anode and separator-wrapped lithium counter electrode with copper conductive layer facing the lithium anode housed in a glass cell for in-situ optical microscopy observation. During charging of the cell, non-uniform deposition of lithium onto the lithium electrode leads to mossy dendrite formation and growth on the surface. ( b ) Voltage profile of the device. The lithium dendrites make contact with the conductive copper layer on the separator at about 6–8 min, giving rise to a 3 V drop in V Cu-Li , as the potential difference between copper and lithium is dissipated on contact. Full size image The stability of the thin metal layer is critical for the successful long-term implementation of our separator design. Therefore, we have examined the durability of the thin metal layer stored in the electrochemical environment of the battery over an extended period of time. Our data confirms that the sheet resistance of the thin metal layer does not show any significant increase ( Supplementary Fig. 12 ). This is certainly not surprising, as copper metal foil is currently used as the anode current collector. In addition, we also show that the voltage between the copper interlayer and lithium metal does not change over a long period during battery storage or battery operation ( Supplementary Figs 13 and 14 ). The copper coating is also stable during cycling and we demonstrate the same dendrite detection capability in a cycled cell with both charging and discharging ( Supplementary Fig. 15 ). This bifunctional separator can also enable the new and exciting possibility of identifying the position of the overgrown dendrite. To demonstrate this, we intentionally created a pinhole in the separator to induce dendrite formation. Once the dendrite forms and bridges the lithium electrode with the copper layer, the location of the corresponding pinhole in one dimension can be determined simply by measuring the resistance between the terminals as illustrated in Fig. 4a . The resistance measured from the separator leads on either end of the copper-coated separator to the negative terminal consists of a fixed copper–lithium junction resistance term, R junc , and a copper sheet resistance term, R 1 or R 2 , which scales with the distance between the pinhole and the two separator leads. R junc can be determined once the resistance between the two separator leads, R 1 + R 2 , is measured. The ratio of the sheet resistances R 1 / R 2 is equivalent to the ratio between the distances from the separator terminals to the pinhole, L 1 / L 2 . The results confirm that this method can accurately detect the dendrite position to within 2% of the actual dendrite position ( Fig. 4b,c ). We emphasize that the dendrite’s growth may occur over a wider area. In that case, the predicted dendrite location will be less accurate, representing only an approximate location of dendrite growth. 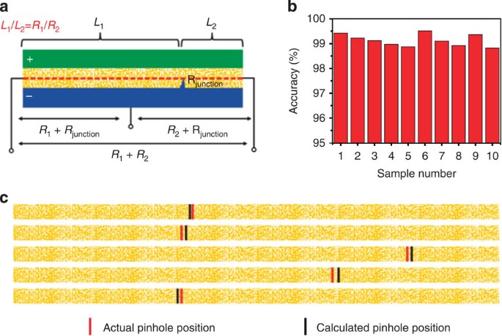Figure 4: Dendrite pinhole puncture position determined by resistance measurement. (a) The resistance measured from the copper-coated separator leads on either side of the separator to the negative electrode lead is made up of a fixed junction resistance term,Rjunc, and a sheet resistance term,R1orR2, which scales with the distance between the pinhole and separator lead.Rjunccan be determined if the resistance between the two separator leads,R1+R2, is measured. The ratio in pinhole position from the two edges of the separator is equivalent to the ratio between the resistances measured between each separator lead and the negative electrode lead. (b) Percentage difference between the actual position and the calculated position of the pinhole from measured resistances and (c) separator schematic indicating relative difference. Figure 4: Dendrite pinhole puncture position determined by resistance measurement. ( a ) The resistance measured from the copper-coated separator leads on either side of the separator to the negative electrode lead is made up of a fixed junction resistance term, R junc , and a sheet resistance term, R 1 or R 2 , which scales with the distance between the pinhole and separator lead. R junc can be determined if the resistance between the two separator leads, R 1 + R 2 , is measured. The ratio in pinhole position from the two edges of the separator is equivalent to the ratio between the resistances measured between each separator lead and the negative electrode lead. ( b ) Percentage difference between the actual position and the calculated position of the pinhole from measured resistances and ( c ) separator schematic indicating relative difference. Full size image Early detection of hazardous conditions allows proactive measures to be implanted to minimize battery failure. Our design and experimental data demonstrate a new simple approach to addressing the safety issues associated with internal short circuiting created during battery charge–discharge and by manufacturing defects. Continuous monitoring of internal operating conditions allows batteries to be operated to the full extent of their lifetime rather than prematurely replacing them in anticipation of possible failure by dendrite overgrowth. Here we would like to have a broader discussion of a variety of features related to this new design. The first feature is related to concerns of reduced energy density of the battery, as the trilayer design might increase the thickness of the separator. We would like to argue here that the intrinsic safety mechanism of detecting dendrite growth half way through the separator before an anode–cathode short is formed will enable the use of much thinner polymer separators on both sides of the metal layer. Thus, ultimately, the total separator thickness will be comparable to or even thinner than the traditional single-layer separator while providing safer operation. Therefore, we believe that the energy density will probably not be reduced with our trilayer design. The second point is whether it is realistic to implement a third electrode connected to the separator in batteries. We believe that it is straightforward to include a third electrode in the pouch cell configuration, although it might be challenging to implement this concept in the cylindrical cell configuration. The third point is on how to produce such a trilayer separator. Even though we demonstrated this concept by stacking two layers of separators with a metal coating between, it is entirely possible to use only one layer of polymer separator as a substrate to deposit the thin metal layer followed by a porous insulating layer, which can be produced by a variety of coating methods such as solution particle coating [22] , gel electrolyte coating [32] , electrospinning of polymer fibres [33] , and copolymer coating and extraction [34] . The fourth feature is that including a third electrode in the battery to detect short circuits opens up new opportunities in battery management systems for much improved control. The fifth is that this battery design concept is generally applicable to other battery types beyond the lithium-based systems discussed herein. Materials fabrication and cell assembly The conducting layer was fabricated by sputtering copper (AJA International ATC Orion, 5 mTorr pressure, 150 W power and 15 s.c.c.m. argon flow) for 5 min onto commercially available 12 μm Teklon Gold LP microporous polyethylene separator membrane. The sheet resistance of the coated separator was determined by applying silver paste lines forming a square on the separator with conducting layer. Electrical measurements were made with a multimeter. Pouch cells with lithium foil as both electrodes were assembled and sealed in an argon-filled glove box. Copper foil was used as electrical leads to the anode and counter electrode as well as the conducting layer. The conducting layer sandwiched between two separators was soaked in electrolyte, 1 M LiPF 6 in ethylene carbonate/diethyl carbonate (1:1; Merck). Electrochemical and electrical test The cells were charged at 4 mA cm −2 , while V Cu-Li was monitored with an MTI eight-channel battery tester. Electrochemical impedance spectroscopy measurements were carried out on a Bio Logic VMP3 with ac oscillation amplitude of 10 mV over the frequency range of 100 kHz to 1 Hz. Separators with varying thicknesses of the conductive layer were soaked in electrolyte and sandwiched between stainless steel electrodes, and then sealed inside a pouch cell. Electrical properties of the separators were measured by an Agilent B1500A semiconductor device analyser. In-situ optical microscopy observation A lithium foil anode and lithium foil counter electrode wrapped in a copper-coated separator were placed facing one another inside a glass observation cell filled with electrolyte. Observation was performed with an Olympus BX51M microscope under normal white-light illumination. Dendrite position detection Copper leads were affixed to both ends of a copper-coated separator and a pinhole was produced by lightly pricking the separator with the tip of a 22-G syringe needle. Assembly of the pouch cell was as outlined previously. The resistances were measured with a multimeter. How to cite this article: Wu, H. et al. Improving battery safety by early detection of internal shorting with a bifunctional separator. Nat. Commun. 5:5193 doi: 10.1038/ncomms6193 (2014).